Magnetic barcode assay for genetic detection of pathogens The task of rapidly identifying patients infected with Mycobacterium tuberculosis in resource-constrained environments remains a challenge. A sensitive and robust platform that does not require bacterial isolation or culture is critical in making informed diagnostic and therapeutic decisions. Here we introduce a platform for the detection of nucleic acids based on a magnetic barcoding strategy. PCR-amplified mycobacterial genes are sequence-specifically captured on microspheres, labelled by magnetic nanoprobes and detected by nuclear magnetic resonance. All components are integrated into a single, small fluidic cartridge for streamlined on-chip operation. We use this platform to detect M. tuberculosis and identify drug-resistance strains from mechanically processed sputum samples within 2.5 h. The specificity of the assay is confirmed by detecting a panel of clinically relevant non- M. tuberculosis bacteria, and the clinical utility is demonstrated by the measurements in M. tuberculosis -positive patient specimens. Combined with portable systems, the magnetic barcode assay holds promise to become a sensitive, high-throughput and low-cost platform for point-of-care diagnostics. Recent advances in genomic profiling have ushered in new opportunities in the diagnosis and treatment of human diseases. Genetic testing has a potential to enable and hasten early disease detection and rationalize treatments, especially in cancer, cardiovascular and infectious diseases [1] , [2] , [3] , [4] . One of the emerging areas of such genetic diagnoses is the detection of tuberculosis (TB). TB is a significant public health threat and economic burden. In 2011, an estimated 8.7 million TB cases were developed with 1.4 million deaths worldwide [5] , [6] . Despite the availability of efficient treatment, controlling the spread of TB remains a challenging task, primarily because of the lack of fast and sensitive detection technology [7] , [8] , [9] . The overall sensitivity of smear microscopy, the most common method for TB diagnosis, is <60%, especially in patients with low bacterial counts (<10,000 ml −1 sputum) or with extrapulmonary disease; bacteria culture is the gold standard in TB detection for its highest sensitivity, but requires weeks to obtain results. Delayed case detection is associated with reduced cure rates and provides opportunity for continued transmission, which became even more a serious problem with the co-infections of HIV and the emergence of highly drug-resistant TB [10] , [11] . Developing a platform for fast, earlier and improved TB detection is thus considered crucial for efficient TB control. Several new TB diagnostic tests have recently been introduced, based on different detection techniques (for example, Gen-Probe RNA test, interferon-gamma assay and urine-based antigen test) [12] , [13] . Nucleic acid amplification tests, in particular, have emerged as a preferred approach for TB detection. The method employs the PCR to amplify a target gene of Mycobacterium tuberculosis (MTB), and thereby enabling high-detection specificity and versatility. The line probe assay, for instance, colorimetrically detects multi-drug-resistant strains from PCR-amplified MTB DNA [14] . Most recently, GeneXpert MTB/rifampin (RIF) (Cepheid) advanced nucleic acid-based detection by integrating PCR and a highly sensitive molecular beacon assay into a single, automated system. Using chemically treated sputum samples, the system detects the presence of MTB as well as RIF-resistance [15] . Implementation of this test, however, is not likely to be feasible in resource-limited and field settings [12] , as the system operation requires the use of sophisticated optics, stable electrical power supply and routine maintenance. We herein report on the development of a nucleic acid platform designed to provide fast and portable detection, and demonstrate the utility by detecting MTB DNA from mechanically processed TB patient sputum samples. The method is based on a magnetic barcoding strategy: PCR-amplified target MTB genes are captured and magnetically labelled by a pair of complementary oligonucleotides conjugated to microspheres and magnetic nanoprobes (MNPs). Combined with portable nuclear magnetic resonance (NMR) systems [16] , [17] , [18] , the assay showed higher sensitivity than smear microscopy, required significantly less time (<2.5 h) than culture methods, and successfully discriminated single-nucleotide polymorphism in target genes, providing facile identification of drug-resistant MTB strains. 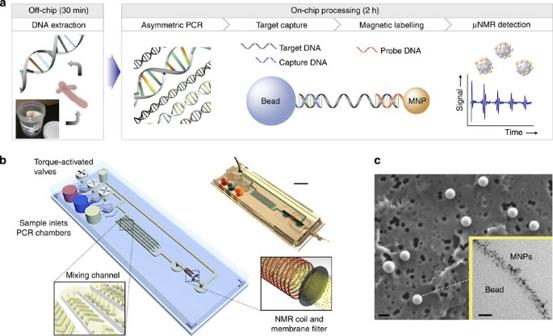Figure 1: Magnetic barcode assay for sensitive TB detection. (a) Assay procedure. From unprocessed sputum specimen, DNA is extracted though an off-chip mechanical stressing. Extracted DNA samples are then loaded into a fluidic device for on-chip processing. The target DNA sequences are amplified by asymmetric PCR and captured by polymer beads modified with capture DNA. MNPs are then used to specifically coat the beads via complementary sequence, and the samples are subjected to NMR measurements. The MNP-labelled beads accelerate the decay of NMR signal, providing analytical signal for nucleic acid detection. The entire assay time is ~2.5 h. (b) A fluidic cartridge was developed to streamline the assay. The device integrates PCR chambers, mixing channels and a microcoil for NMR measurements. The entire system was designed as a disposable unit to prevent cross-contamination of PCR-amplified products. Whole-genomic DNA, extracted from expectorated samples, capture beads and MNPs are loaded into inlet chambers gated by screw valves. After on-chip PCR, magnetic labelling of the beads takes place along the mixing channel. The magnetically barcoded beads are then purified and concentrated into the μNMR probe (microcoil) by the membrane filter. Scale bar, 1 cm. (c) Scanning electron microscopy confirmed the bead capture by the membrane filter. Scale bar, 1 μm. Transmission electron microscopy revealed that beads are efficiently labelled with MNPs (inset). Scale bar, 30 nm. Magnetic barcode platform for MTB detection Figure 1a illustrates the magnetic barcode assay, designed to detect mycobacterial nucleic acids. In the current prototype, sputum samples are first processed off-chip to extract DNA from MTB. We adopted a simple mechanical method based on vigorous mixing with glass beads. Following the DNA extraction, the target DNA region is amplified through PCR. The amplicons are captured on polymeric beads (diameter: 1 μm) modified with complementary capture DNAs. Subsequently, the beads are rendered superparamagnetic by coupling MNPs (30 nm) to the opposite end of the amplicon. This scheme enhances detection specificity through the simultaneous tagging by the capture and the probe DNAs; it also offers fast binding kinetics (<1 min) as the labelling is performed in a small sample volume. The magnetic nanoparticles contain iron oxide cores encased by heat-resistant crosslinked dextran shells, to ensure high stability in varying salt conditions and the required nucleotide-annealing temperatures. After removing excess MNPs, samples are subject to NMR measurements. MNP-loaded beads produce local magnetic fields, which lead to faster relaxation of the 1 H NMR signal. The decay rate is proportional to the MNP concentration (and thus initial DNA), enabling quantification of target DNAs. Figure 1: Magnetic barcode assay for sensitive TB detection. ( a ) Assay procedure. From unprocessed sputum specimen, DNA is extracted though an off-chip mechanical stressing. Extracted DNA samples are then loaded into a fluidic device for on-chip processing. The target DNA sequences are amplified by asymmetric PCR and captured by polymer beads modified with capture DNA. MNPs are then used to specifically coat the beads via complementary sequence, and the samples are subjected to NMR measurements. The MNP-labelled beads accelerate the decay of NMR signal, providing analytical signal for nucleic acid detection. The entire assay time is ~2.5 h. ( b ) A fluidic cartridge was developed to streamline the assay. The device integrates PCR chambers, mixing channels and a microcoil for NMR measurements. The entire system was designed as a disposable unit to prevent cross-contamination of PCR-amplified products. Whole-genomic DNA, extracted from expectorated samples, capture beads and MNPs are loaded into inlet chambers gated by screw valves. After on-chip PCR, magnetic labelling of the beads takes place along the mixing channel. The magnetically barcoded beads are then purified and concentrated into the μNMR probe (microcoil) by the membrane filter. Scale bar, 1 cm. ( c ) Scanning electron microscopy confirmed the bead capture by the membrane filter. Scale bar, 1 μm. Transmission electron microscopy revealed that beads are efficiently labelled with MNPs (inset). Scale bar, 30 nm. Full size image To streamline the assay procedure, we developed a microfluidic device for on-chip magnetic barcode assay ( Fig. 1b ). The device performs key functions of the assay: PCR amplification, magnetic labelling and NMR measurements ( Supplementary Fig. S1 ). The assay uses sputum samples that are mechanically liquefied and loaded into the on-chip PCR chambers along with PCR reagents. MNPs and buffer solutions are loaded into separate chambers gated by valves. After target DNA sequences are PCR-amplified, the PCR products are combined with capture beads. The bead-DNA mixture and MNPs are then introduced into the extended mixing channel. The MNPs would only bind to the capture beads in the presence of the target amplicons. The MNP-labelled beads are purified by an in-line membrane filter ( Fig. 1c ) and concentrated into the miniaturized NMR (μNMR) chamber for detection (see Methods for detailed fluidic operations). Custom-designed portable NMR electronics are used to monitor and compensate for temperature drifts, which enables robust measurements across different temperature environments (4–50 °C) [17] . Assay optimization We first optimized the assay protocol to maximize the magnetic signal. Samples were prepared using synthetic 92-nucleotide (nt) single-stranded DNA (ssDNA) specifically found within the acyl-CoA dehydrogenase fadE15 gene of MTB [19] , [20] . Non-complementary 92-nt ssDNA was used for control samples. The transverse relaxation rate ( R 2 ) of samples was measured, and the magnetic signal was defined as R 2 ratio between the target and the control samples (see Methods for details). When ssDNA and double-stranded DNA samples were compared ( Supplementary Fig. S2a ), ssDNA displayed higher signal; double-stranded DNA required additional denaturing and annealing steps, which lowered the binding stability of capture beads and MNP probes. For the ssDNA samples, the highest signal could be obtained when the target ssDNA was first captured by beads and then labelled with MNPs; this approach presumably minimized competitive binding to ssDNA between capture beads and MNPs [21] . Based on these results, we adopted the asymmetric PCR and sequential labelling strategy for target DNA production and its magnetic targeting, respectively. The assay conditions for sequential labelling were further refined ( Supplementary Fig. S2b ). Four different sizes of capture beads ranging from 0.5 to 5 μm were tested to determine the most efficient substrate for DNA capture. After the capture beads were incubated in the ssDNA solution and labelled with MNPs, NMR measurements were performed under the same weight concentration for each bead size. The 1-μm capture beads provided not only large surface area for capturing and magnetic labelling but also had the lowest nonspecific binding, which resulted in the highest magnetic signal. The optimal incubation temperature was ~37 °C, agreeing with the melting temperature ( t m =45 °C) of 92-nt fadE15 amplicons estimated by hairpin analysis [22] . With each MNP conjugated with >50 probe strands, the magnetic labelling of beads could be completed in <1 min, benefiting from the multiple binding valency of MNPs. The developed assay protocol was applied to detect 92-nt segment of fadE15 ssDNA ( Fig. 2a ). Fluorescence imaging showed strong co-localization of the near-infrared fluorescent MNPs with green-fluorescent capture beads ( Fig. 2b ). Flow-cytometry analysis further showed highly specific MNP labelling on beads only in the presence of target ssDNA ( Fig. 2c ). On-chip μNMR measurements confirmed the specific detection of the target ssDNA ( Fig. 2d ) with similar signal-to-noise ratio as in flow cytometry. Note that the μNMR required much lower number of beads: ~10 6 beads in 1 μl volume compared with ~10 9 beads in 250 μl volume for flow cytometry. The sequence-specific hybridization between oligonucleotides further enabled highly selective amplification of MNP loading onto the bead surface, offering versatility in magnetic labelling. For example, by applying a pair of MNPs conjugated with complementary oligonucleotide sequences, we could form multiple MNP layers and thus amplified particle loading onto beads ( Fig. 2e , left). The resulting NMR signal for target samples increased by nearly threefold, whereas control samples showed negligible increase in identically treated beads using non-complementary ssDNA ( Fig. 2e , right). 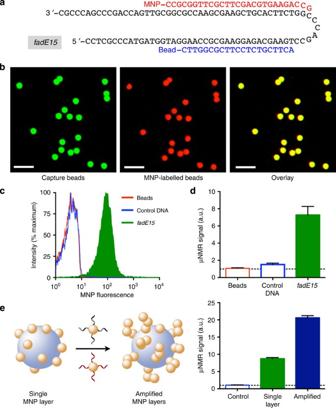Figure 2: Assay optimization and amplification process. (a) A segment (92-nt) offadE15ssDNA was used as a detection target. Capture beads and MNPs were conjugated with complementary oligonucleotides. (b) Following on-chip labelling, confocal microscopy of the magnetically barcoded beads were performed. The fluorescent polystyrene beads (green) co-localized with the near-IR fluorescence of the MNPs (red) in the presence of targetfadE15ssDNA. Scale bar, 5 μm. (c) Measurements by flow cytometry confirmed target-specific labelling of the beads. Non-complementary ssDNA samples showed low signal close to that of control. (d) Corresponding μNMR detection also displayed strong signal with the presence offadE15amplicons. (e) Sequential layering of the capture beads was performed using MNPs conjugated to alternating oligonucleotide sequences. Such layering amplified the number of MNP probes on the bead surface and therefore increased the overall magnetic signal. The error bars indanderepresent the s.d. of three replicates (n=3). Figure 2: Assay optimization and amplification process. ( a ) A segment (92-nt) of fadE15 ssDNA was used as a detection target. Capture beads and MNPs were conjugated with complementary oligonucleotides. ( b ) Following on-chip labelling, confocal microscopy of the magnetically barcoded beads were performed. The fluorescent polystyrene beads (green) co-localized with the near-IR fluorescence of the MNPs (red) in the presence of target fadE15 ssDNA. Scale bar, 5 μm. ( c ) Measurements by flow cytometry confirmed target-specific labelling of the beads. Non-complementary ssDNA samples showed low signal close to that of control. ( d ) Corresponding μNMR detection also displayed strong signal with the presence of fadE15 amplicons. ( e ) Sequential layering of the capture beads was performed using MNPs conjugated to alternating oligonucleotide sequences. Such layering amplified the number of MNP probes on the bead surface and therefore increased the overall magnetic signal. The error bars in d and e represent the s.d. of three replicates ( n =3). Full size image Detection sensitivity and specificity The sensitivity of the magnetic barcode platform was comprehensively characterized using samples in different formats. We first used serially diluted fadE15 ssDNA samples, and determined the absolute detection limit of the magnetic barcode assay; without the PCR amplification step, the detection limit was ~1 nM ssDNA in 1 μl sample volume ( Fig. 3 ). We next loaded genomic MTB DNA into the device, amplified the 92-nt segment of fadE15 via asymmetric PCR and performed the magnetic barcode assay. With PCR amplification of the target gene, the system could detect down to 1–5 genomic DNA in buffer solution ( Fig. 4a ), demonstrating the potential to detect a single bacterium. 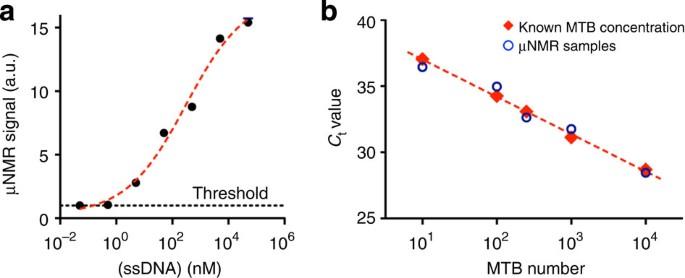Figure 3: Titration assay and PCR characterization of MTB genomic DNA. (a) The detection sensitivity of the magnetic barcode assay without PCR amplification was determined. Samples containing 92-ntfadE15ssDNA were serially diluted and magnetically labelled. The detection limit was ~1 nM of ssDNA in 1 μl sample volume. The error bars inarepresent the s.d. of three replicates (n=3). (b) Real-time PCR was used to correlate the amount of genomic DNA and to determine the detection sensitivity. Number of genomic copies was estimated using mass calculation, assuming molecular weight of 660 per base pair and MTB genome size of 4411529. Serial dilution of genomic DNA sample was performed to establish reverse transcription-PCR standard. Separate genomic DNA dilution was performed to contain 1, 10, 25, 100 and 1000 genome, and Ct values of the samples were compared with the standard. The sample dilution was used for μNMR measurements. Figure 3: Titration assay and PCR characterization of MTB genomic DNA. ( a ) The detection sensitivity of the magnetic barcode assay without PCR amplification was determined. Samples containing 92-nt fadE15 ssDNA were serially diluted and magnetically labelled. The detection limit was ~1 nM of ssDNA in 1 μl sample volume. The error bars in a represent the s.d. of three replicates ( n =3). ( b ) Real-time PCR was used to correlate the amount of genomic DNA and to determine the detection sensitivity. Number of genomic copies was estimated using mass calculation, assuming molecular weight of 660 per base pair and MTB genome size of 4411529. Serial dilution of genomic DNA sample was performed to establish reverse transcription-PCR standard. Separate genomic DNA dilution was performed to contain 1, 10, 25, 100 and 1000 genome, and Ct values of the samples were compared with the standard. The sample dilution was used for μNMR measurements. 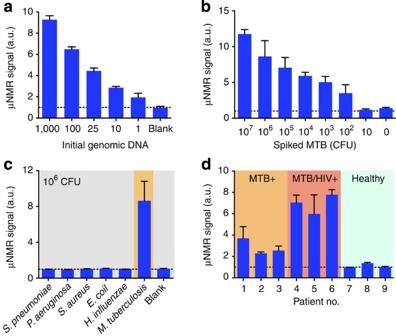Figure 4: MTB detection sensitivity using the magnetic barcode assay. (a) The detection limit of the platform with PCR steps was established. Genomic MTB DNA was loaded on the fluidic chip, and the 92-nt segment offadE15amplicons were prepared by asymmetric PCR. Titration experiments with initial DNA loading showed that the assay could detect down to a few genomic DNA in buffer solution. (b) Detection of MTB within sputum samples. Whole MTB cells were spiked into 0.5 ml aliquots of MTB-negative sputa to the final concentrations ranging from 0–107CFU ml−1. Following the off-chip DNA extraction, samples were measured by the magnetic barcode assay. The sensitivity was 102−103CFU ml−1. (c) Control samples containing non-MTB bacteria (106CFU ml−1) spiked into the sputa were used to confirm the specificity of the primers and barcode assay. Samples measured from the non-MTB controls displayed baseline magnetic signal, similar to the blank sputa in which no MTB was present. (d) Clinical sputum specimens were analysed with the μNMR assay. Compared with the samples collected from MTB-positive patients, the samples collected from MTB/HIV-positive patients showed higher μNMR signals. MTB-negative sputa collected from healthy volunteers were used as negative controls. The error bars ina–drepresent the s.d. from triplicate measurements. Full size image Figure 4: MTB detection sensitivity using the magnetic barcode assay. ( a ) The detection limit of the platform with PCR steps was established. Genomic MTB DNA was loaded on the fluidic chip, and the 92-nt segment of fadE15 amplicons were prepared by asymmetric PCR. Titration experiments with initial DNA loading showed that the assay could detect down to a few genomic DNA in buffer solution. ( b ) Detection of MTB within sputum samples. Whole MTB cells were spiked into 0.5 ml aliquots of MTB-negative sputa to the final concentrations ranging from 0–10 7 CFU ml −1 . Following the off-chip DNA extraction, samples were measured by the magnetic barcode assay. The sensitivity was 10 2 −10 3 CFU ml −1 . ( c ) Control samples containing non-MTB bacteria (10 6 CFU ml −1 ) spiked into the sputa were used to confirm the specificity of the primers and barcode assay. Samples measured from the non-MTB controls displayed baseline magnetic signal, similar to the blank sputa in which no MTB was present. ( d ) Clinical sputum specimens were analysed with the μNMR assay. Compared with the samples collected from MTB-positive patients, the samples collected from MTB/HIV-positive patients showed higher μNMR signals. MTB-negative sputa collected from healthy volunteers were used as negative controls. The error bars in a – d represent the s.d. from triplicate measurements. Full size image To evaluate the overall detection sensitivity, we used sputum samples spiked with live MTB. To mimic clinical cases, we varied the final MTB concentration up to 10 7 colony forming unit (CFU) ml −1 . Genomic DNA was first released off-chip through the mechanical disruption, and divided into two aliquots. The first half was used for conventional real-time PCR ( Fig. 3b ). The other half was processed by the magnetic barcode device; after the asymmetric PCR of 92-nt fadE15 , we introduced capture beads into the PCR chamber to capture the amplicons, and then magnetically labelled the beads along the microfluidic channel. Titration measurements established that the detection limit was ~10 3 spiked MTB in 1 ml sputum ( Fig. 4b ). The observed sensitivity was lower than with pure genomic DNA samples. This could be attributed to suboptimal DNA extraction with spiked samples. Additional sample loss presumably happened during the off-chip DNA extraction and transfer processes. The current magnetic barcoding assay, however, was superior to smear test (detection threshold ~10 4 CFU in 1 ml of sputum) and was considerably faster (2.5 h) than culture-based method that requires weeks [23] , [24] . To improve the sensitivity, we intend to combine the mechanical extraction process with chemical treatment and DNA purification. Note that the barcode assay also showed a good correlation with separate real-time PCR of whole-genomic extracts ( Fig. 3b ). Signals from sputum samples containing high concentration (10 6 CFU ml −1 ) of clinically relevant non-MTB species ( Streptococcus pneumoniae , Pseudomonas aeruginosa , Staphylococcus aureus , Escherichia coli and Haemophilus influenzae ) were nearly identical to those from control sputa ( Fig. 4c ), indicating that nonspecific amplification and/or binding of the primers was negligible. Such high specificity would be crucial to achieve accurate MTB detection from complex specimens, which may contain multiple bacterial strains. TB detection in clinical samples To evaluate the clinical utility of the magnetic barcode platform, we analysed clinical sputum samples from MTB smear-positive patients, and as a negative control, sputa from healthy patients without a diagnosis of MTB infection. The magnetic barcode assay detected the presence of MTB in all MTB-positive patient samples ( Fig. 4d ). With control samples, the signal was at the baseline level, confirming the specificity of the assay. Interestingly, the assay performed well in patients with MTB/HIV co-infection. Diagnostics for these patients remain unclear because the standard approaches often perform poorly, yet studies have shown that HIV co-infection induces greater bacterial burden by accelerating the growth of MTB [11] , [25] , [26] . This finding supports our measurement of a higher bacterial burden in co-infected patient sputum. Analysis of single-nucleotide mutation Drug-resistant TB strains can be detected by identifying specific genetic mutations. For instance, over 95% of RIF-resistant MTB strains have mutations within the 81-nt core region of the rpoB gene ( Fig. 5a , top), whereas the mutation is absent in nearly all RIF-susceptible strains [2] . Approximately 90% of RIF-resistant MTB is also resistant to isoniazid, which makes the mutant rpoB gene as a potential surrogate marker for multi-drug-resistant TB [27] . 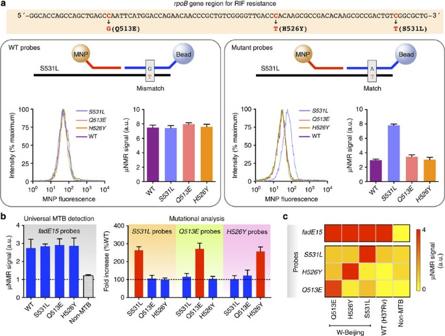Figure 5: Magnetic detection of single-nucleotide polymorphism. (a) Magnetic barcode assay was optimized to detect point mutations inrpoBgene (Q513E, C-to-G; H526Y, C-to-T; S531L, C-to-T), which confer drug (RIF) resistance to MTB. When the capture beads are complementary to therpoBWT ssDNA, both fluorescence and magnetic readouts were indiscernible amongrpoBalleles (left). When the capture DNA sequence was modified to fully match the single-nucleotide polymorphism in S531L-mutant strand, the magnetic barcode assay could selectively detect the target gene (right). (b) The optimized set of magnetic barcode probes (Supplementary Fig. S5a) could effectively detect the presence of MTB (viafad15Eprobes) as well as analyse the mutational status (viarpoBprobes). For each probe, the signal levels were normalized against that of a WT sample. The data inaandbare displayed as mean±s.d. from triplicate measurements. (c) Magnetic profiling on a panel of MTB strains in sputum samples. RIF-resistant W-Beijing strains, and WT H37Rv strains were spiked in sputa (104CFU ml−1); non-MTB mixed bacteria was used as the control. Following the DNA extraction, samples were loaded onto the device for PCR and magnetically labelled. The heat map showed the universal MTB detection using thefadE15probes, as well as the sequence-specific identification of RIF-resistance with therpoBprobes. Figure 5: Magnetic detection of single-nucleotide polymorphism. ( a ) Magnetic barcode assay was optimized to detect point mutations in rpoB gene (Q513E, C-to-G; H526Y, C-to-T; S531L, C-to-T), which confer drug (RIF) resistance to MTB. When the capture beads are complementary to the rpoB WT ssDNA, both fluorescence and magnetic readouts were indiscernible among rpoB alleles (left). When the capture DNA sequence was modified to fully match the single-nucleotide polymorphism in S531L-mutant strand, the magnetic barcode assay could selectively detect the target gene (right). ( b ) The optimized set of magnetic barcode probes ( Supplementary Fig. S5a ) could effectively detect the presence of MTB (via fad15E probes) as well as analyse the mutational status (via rpoB probes). For each probe, the signal levels were normalized against that of a WT sample. The data in a and b are displayed as mean±s.d. from triplicate measurements. ( c ) Magnetic profiling on a panel of MTB strains in sputum samples. RIF-resistant W-Beijing strains, and WT H37Rv strains were spiked in sputa (10 4 CFU ml −1 ); non-MTB mixed bacteria was used as the control. Following the DNA extraction, samples were loaded onto the device for PCR and magnetically labelled. The heat map showed the universal MTB detection using the fadE15 probes, as well as the sequence-specific identification of RIF-resistance with the rpoB probes. Full size image We set out to optimize the magnetic barcode assay for fast detection of single-nucleotide polymorphism on the segments of the rpoB gene. We initially focused on detecting the C-to-T mutation in codon 531 (S531L), which is the most common amino-acid substitution responsible for RIF resistance. This mutation is observed in 70% of drug-resistant strains found in the clinics [14] , and these strains are reported to be the most transmissible and have the highest fitness level (that is, survival under pressure) [28] . Two types of capture 20-nt oligonucleotide for the rpoB amplicons were designed, one fully complementary to wild-type (WT) strand and the other to the S531L-mutant strand. The 81-nt rpoB ssDNA assumed a high hairpin melting temperature at ~68 °C (ref. 22 ), requiring higher incubation temperate (60 °C) during the magnetic labelling. With the WT-capture beads, the barcode assay universally detected rpoB strands regardless of their mutational status ( Fig. 5a , left). Capture beads that fully complement with S531L mutation, on the other hand, were able to distinguish the specific mutation ( Fig. 5a , right); magnetic signals were >400% higher with S531L-mutant strands than with WT or other rpoB mutant strands (Q513E, C-to-G mutation in codon 513; H526Y, C-to-T mutation in codon 526). Interestingly, when a similar strategy was applied to the MNPs, that is, having the oligonucleotide on the MNPs match the mutant rpoB ssDNA, no difference in binding affinity was observed between the target mutant and other strands ( Supplementary Fig. S3 ). It is likely that the multiple binding valency of MNPs resulted in higher binding affinity with the rpoB strands and prevented the discrimination of the single-nucleotide mismatch [29] . Capture oligonucleotides probes were further developed to detect other rpoB mutations that lead to clinically relevant amino-acid substitutions, H526Y and Q513E. Unlike the case with S531L, initial 20-nt probes for H526Y and Q513E were ineffective in discriminating target mutant strands ( Supplementary Fig. S4 ). Analysis of the rpoB ssDNA revealed that the binding region for the S531L capture probe contains higher G/C contents and forms stable hairpin structure ( t m =80 °C), whereas Q513E and H526Y regions have less stable hairpin structure ( t m =50–60 °C). We thus hypothesized that reducing the length of capture probes would improve the specificity to Q513E and H526Y by decreasing the thermodynamic stability for single-nucleotide mismatch binding. Indeed, when the capture sequence was reduced to 15 nt, high selectivity for corresponding mutant strands could be achieved ( Supplementary Fig. S4 ). These probes displayed consistent, high signal-to-noise ratios (~300%) and complemented the fadE15 probe for comprehensive MTB analyses ( Fig. 5b ). We finally tested the developed platform to detect RIF-resistant and WT strains of MTB. RIF-resistant MTB colonies were cultured and screened for specific rpoB mutations through sequencing. Samples were prepared by spiking MTB in sputa. Extracted DNA samples were amplified for 126-nt segment of rpoB and 92-nt segment of fadE15 regions, followed by the labelling with the optimized probe set ( Supplementary Fig. S5a ). Although the WT strain yielded only positive signal for the fadE15 probes, the Q513E, H526 and S531L-mutant isolates yielded positive signals for both the fadE15 and the corresponding mutant rpoB probes ( Fig. 5c and Supplementary Fig. S5b ). We further profiled a mixed population of WT and RIF-resistant strains ( Fig. 6 ). Through multi-channelled measurements using both WT and mutant-specific probes, we could determine the ratio between RIF-resistance and susceptible MTB; such a capacity could potentially be used to study the bacterial mutation rate in culture during antibiotic treatments [30] . One of the methods that could be implemented to detect low ratios of resistant strain in mixed population would be to combine the magnetic barcode assay with droplet-based PCR. 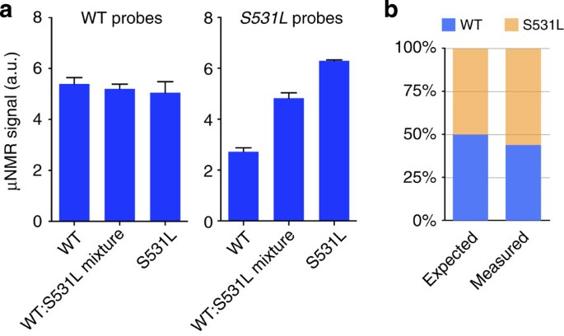Figure 6: Analysis of heterogeneous strain mixture. (a) By using the probe sequences and assay described inSupplementary Fig. S5, the 1:1 mixture of mutant S531L isolates and drug-susceptible strain (106CFU for each strain) could be detected by the magnetic barcode assay. All measurements are in triplicate, and the data are shown as mean±s.d. (b) The ratio between WT and S531L population was obtained froma. The measured ratio (WT/S531L=56/44) was close to the expected value (50/50). [31] Figure 6: Analysis of heterogeneous strain mixture. ( a ) By using the probe sequences and assay described in Supplementary Fig. S5 , the 1:1 mixture of mutant S531L isolates and drug-susceptible strain (10 6 CFU for each strain) could be detected by the magnetic barcode assay. All measurements are in triplicate, and the data are shown as mean±s.d. ( b ) The ratio between WT and S531L population was obtained from a . The measured ratio (WT/S531L=56/44) was close to the expected value (50/50). Full size image We have developed a new magnetic assay system for fast and facile detection of MTB. The use of magnetic detection considerably simplifies the assay and system design. Magnetic assays experience little interference from biological matrices and thus can be performed on crude specimens without extensive purification steps. Unlike optical systems, the measurement setup can be easily packaged as a miniaturized, portable electronics. Indeed, we have integrated PCR, fluidics and NMR probes into a single fluidic cartridge (2.5 × 7.5 cm 2 , the size of a standard microscope slide) for streamlined on-chip operations. Furthermore, we have systematically optimized the magnetic barcode probes to maximize detection sensitivity and specificity. The platform has many innovative features, presenting a new multidisciplinary approach to TB diagnosis. First, the magnetic barcoding strategy enhances detection specificity and sensitivity through double-targeting (capture and labelling probes) and magnetic layering, respectively. Importantly, the method also detects single-gene mutations, which enables simultaneous identification of drug-resistance MTB strains. This is a significant advance from our previous approach that utilized antibody-conjugated MNPs to target bacteria (Bacillus Calmette–Guérin as MTB surrogate) [18] ; the method is limited by the specificity of antibodies and unable to identify drug-resistant strains. Second, the integrated fluidic cartridge, which combines on-chip PCR and in-line NMR detection, streamlines the assay procedure as well as minimizes sample loss and contamination. The use of μNMR detection further simplifies the assay, as crude DNA extracts can be directly used. These are key factors that allowed fast MTB detection and mutational analyses (2.5 h) from minimally processed sputum samples. Third, the assay system is designed for ultimate applications in point-of-care clinical settings. The miniature μNMR electronics is capable of robust measurements in a wide range of environmental temperature [17] . The assay readout is numerical data ( R 2 ) that requires little interpretation by operators; it can be further simplified as a binary report (positive/negative) for point-of-care applications. The assay platform is affordable for routine use as well. The one-time cost for the equipment, including the sputum processing and readout systems, is about US$4,300, and the assay cost is under US$3 for a fluidic device and chemical reagents ( Supplementary Note 1 ). The magnetic barcode platform is a versatile technology that could be readily applied to other studies and diseases. By changing the probe sequences, it could be a first-response tool to detect pathogens in hospital-acquired infections, food chains and biodefense. The system could also be a bedside tool to identify genetic mutations in chronic diseases, including cancer, heart diseases and diabetes. As an example, we applied the platform to detect the single-point mutation in exon 21 of epidermal growth factor receptor ( Supplementary Fig. S6 ), which has clinical implications in lung cancer [32] . The barcoding strategy is not limited to magnetic readout, but can be extended to luminescent and plasmonic readouts using quantum dots and gold nanoprobes, respectively [33] . Indeed, these methods can be used to simultaneously probe multiple target strands with the arrayed colours of quantum dots and surface-enhanced Raman dyes ( Supplementary Fig. S7 ) [34] . The current prototype is being further improved for more robust operation in resource-limited settings. Most important, we are developing a fluidic device for an initial sample processing. Based on inertial focusing and chemical extraction [35] , [36] , this device is designed to allow direct, high-throughput DNA extraction from sputum samples, replacing the current mechanical setup. We envision the ultimate integration of DNA extraction and detection into a single chip, to provide one-step TB detection. Such a system will further minimize assay time, potentially enabling TB diagnosis and treatment decision at a single visit. Other areas of improvements include the use of loop-mediated isothermal amplification and replication protein A to increase the amplicon yield as well as eliminate the temperature cycling steps [37] , [38] , and combining the electronics with a wireless device would enable efficient data storage and sharing between central laboratories and remote clinics for real-time disease control. With these features, the magnetic barcode assay would then be a truly enabling technology for point-of-care diagnostics. Device fabrication Microfluidic devices were fabricated in polydimethylsiloxane (PDMS) (Dow Corning) using soft lithography [39] . As a channel mould, we patterned two layers of epoxy-based SU8-3050 photoresist (Microchem) on silicon wafers using conventional photolithography. The channel patterns were cast into a 1-mm thick PDMS layer. Separately, we prepared a PDMS block embedded with a microcoil and a membrane filter (400 nm, Nuclepore; Whatman) [18] . The coil block and torque-actuated valves (bolt-nut pairs) [40] were then glued at designated areas on the cured 1-mm PDMS layer, and another 3-mm thick PDMS was poured on the assembly. After curing, fluidic ports were punched out, and the final PDMS layer was irreversibly bonded to a glass slide. Synthesis of capture beads and MNPs All oligonucleotides were purchased from Integrated DNA Technologies. The list of oligonucleotides used in the experiments are summarized in Supplementary Methods . To prepare the capture beads, 500 μg streptavidin-coated polystyrene microbeads (1 μm, 8 × 10 8 beads; Spherotech) were incubated in 50 μl Tris-B (20 mM Tris, pH 7.5, 1 M NaCl, 1 mM EDTA and 0.0005% Triton X-100) containing biotinylated capture DNA (1 nmol) for 30 min at room temperature and then purified. Crosslinked dextran-coated iron oxide particles (CLIO-47) were used for the magnetic labelling of beads. These particles are approximately 30 nm in hydrodynamic diameter (3 nm iron oxide core) and have an R 2 relaxivity value of 70 mM −1 [Fe] s −1 . The synthesis of amine-terminated probes and their conjugation with fluorescent molecules (fluorescein isothiocyanate, AF568 and VT680) were both done using a previously described protocol [41] . Each fluorescent conjugate had 5–8 dye molecules as well as 90 amine groups for further conjugation. To attach oligonucleotides to the probe, MNPs (0.25 mg) were first mixed with sulfo-SMCC (180 μg) in 0.625 ml PBS solution (pH 7.2) for 3 h. Meanwhile, thiol-modified oligonucleotides (40 nmol) were mixed with dithiothreitol (0.1 M) in 100 μl PBS (1 mM EDTA, pH 8) for 2 h. The reduced oligonucleotides were then purified using a NAP-5 column (GE Healthcare), with deionized water as the eluent solution. Absorbance measurements were used to determine the fractions containing the reduced oligonucleotides and the bicinchoninic protein assay solution (Thermo Fisher Scientific) was used to determine the fractions containing dithiothreitol. MNP-SMCCs were subsequently purified using membrane filtration (MWCO 30,000; Millipore Amicon) and Sephadex G-50 (GE Healthcare) with PBS as the eluent buffer. The purified maleimide-activated MNPs were eventually mixed with the reduced oligonucleotides in 2 ml PBS solution (pH 7.2) and the reaction proceeded overnight at room temperature. After this incubation, the conjugates were purified using membrane filtration (MWCO 100,000; Millipore Amicon) and Sephadex G-100 with PBS as the eluent buffer. Conjugation with 6-carboxyfluorescein-modified oligonucleotides was used to confirm that approximately 50 oligonucleotides were conjugated to each MNP. Bacteria culture The risk of infection by MTB is significantly higher for workers handling live bacteria. Infections are typically caused by the production of aerosols containing MTB. Therefore, safety precautions in the handling of MTB inside the Biosafety Level (BSL) 3 laboratories should combine administrative controls, containment principles, laboratory practices, safety equipment and proper facilities. Protective clothing, gloves, eye protection and respiratory protection are required for all experiments inside the BSL 3 laboratories. MTB isolates/strains H37Rv were grown under standard growth conditions at 37 °C with shaking to an optical density (OD)=1.0 in Middlebrook 7H9 broth supplemented with oleic acid, albumin, dextrose, catalase (BBL Middlebrook OADC Enrichment), 0.0005% Tween 80 and 0.2% glycerol. RIF-resistant strains were prepared using clinical W-Beijing strains. Twenty independent cultures were grown in 7H9 broth supplemented with OADC, 0.05% Tween 80 and 0.5% glycerol. Cultures were grown at 37 °C to an OD=1.2. These independent cultures were plated onto 7H10 plates supplemented with OADC, 0.05% Tween 80, 0.5% glycerol and 2 μg ml −1 of RIF. After 28 days of incubation at 37 °C, mutants were randomly selected and analysed via PCRs (forward primer: TCGGCGAGCTGATCCAAAACCA; reverse primer: ACGTCCATGTAGTCCACCTCAGA). PCR products were purified and sequenced via Sanger sequencing methods. Sequencing data revealed specific nucleotide mutations in the rpoB region, the gene encoding for RNA polymerase subunit B. Specific mutants were chosen from each strain for further experiments. Clinical specimens The patient sputum samples were collected in Dar Es Salaam, Tanzania, under a grant from the Bill and Melinda Gates Foundation as part of Grand Challenge 13. The study was approved by the Harvard School of Public Health, and the Broad Institute of Harvard and MIT Institutional Review Board (IRB Protocol No. 18877-102). Subjects had a persistent cough for 2–3 weeks and a confirmed diagnosis of TB based on positive smear microscopy and culture results. Within a BSL 3 laboratory setting, the specimens were mechanically processed as described above to release the genomic DNA. The samples were then aliquoted into a 96-well plate to be baked at 80 °C to ensure the safety of handling. A volume of 10 μl of the sample was used for PCR amplification. The PCR amplification and sample measurements of the processed samples followed similar procedure as described above. The handling of these specimens followed all necessary safety precautions inside the BSL 3 laboratory. PCR for DNA amplification MTB were resuspended in PBS and the concentration was determined by measuring the sample OD. These bacteria were spiked into 0.5 ml aliquots of MTB-negative discarded sputum samples to a final concentration of 0–10 7 CFU ml −1 . Genomic DNA was mechanically released by adding 250 μl of glass beads (0.1 mm diameter) and stressing the sample with FastPrep-24 Instrument (MP Biomedicals) at 50 s pulse with three intervals. Samples were incubated on ice between intervals. The samples then underwent heat treatment to ensure the safety of handling. In a typical PCR reaction, each chamber on the device contained: 0.4 μM of primers, 25 μl of PCR Mastermix (Promega, 400 μM dNTP, 3 mM MgCl 2 and Taq DNA polymerase) and 1–10 μl of spiked sputum (mechanically stressed). PCR-grade water was used to bring the reaction volume to 50 μl. PCR conditions were maintained at 95 °C for 10 min before initiation of 50 cycles: denaturing (95 °C for 30 s), annealing (60 °C for 30 s) and extending (72 °C for 30 s). fadE15 Primer-1 and fadE15 Primer-2 were used for the identification of MTB; rpoB Primer-1 and rpoB Primer-2 were used for the identification of RIF resistance. Primer-1/Primer-2 at a ratio of 10:1 ratio was used for the asymmetric PCR reaction to produce excess single-stranded oligonucleotide (ssDNA) products. On-chip magnetic barcoding assay During the PCR step, all of the valves were closed. After completion of PCR step, 1 μg capture beads (1.6 × 10 6 beads) were mixed with the 50 μl PCR product mixture for 3 min (37 °C for fadE15 assays; 60 °C for rpoB assays). The buffer inlet containing complete PBS (CPBS; 1 × PBS with 1% FBS and 2% BSA) was opened, and the channels were filled with CPBS by pulling from the syringe pump on the outlet. After opening the inlet valves containing the capture beads, PCR product mixture and the MNPs (50 μl, 20 μg ml −1 ), the syringe pump on the outlet was pulled again to mix the reagents. The microbeads were captured and purified on the membrane filter. The buffer inlet was filled with more CPBS to complete the washing process. Following the washing, the flow was gently reversed (10 μl min −1 ) to release the beads from the membrane filter. Changes in the transverse relaxation rate (Δ R 2 ) were measured using a μNMR electronics [16] . The sample volume per measurement was 1 μl. Carr–Purcell–Meiboom–Gill pulse sequences with the following parameters were used; echo time, 4 ms; repetition time, 6 s; the number of 180° pulses per scan, 500; and the number of scans, 8. All measurements were performed in triplicate, and the data are presented as mean±s.e. The measured Δ R 2 value is proportional to the number of MNPs per bead. The NMR signal was obtained from Δ R 2 =Δ R 2 sample /Δ R 2 ø , where Δ R 2 sample and Δ R 2 ø are the relaxation rates for the target sample and control samples, respectively. Flow-cytometry measurements were performed using a BD LSR II flow cytometer, and the mean fluorescence intensity was determined using FlowJo software. How to cite this article: Liong, M. et al . Magnetic barcode assay for genetic detection of pathogens. Nat. Commun. 4:1752 doi: 10.1038/ncomms2745 (2013).